Enzyme activity in liquid lipase melts as a step towards solvent-free biology at 150 °C Water molecules play a number of critical roles in enzyme catalysis, including mass transfer of substrates and products, nucleophilicity and proton transfer at the active site, and solvent shell-mediated dynamics for accessing catalytically competent conformations. The pervasiveness of water in enzymolysis therefore raises the question concerning whether biocatalysis can be undertaken in the absence of a protein hydration shell. Lipase-mediated catalysis has been undertaken with reagent-based solvents and lyophilized powders, but there are no examples of molecularly dispersed enzymes that catalyse reactions at sub-solvation levels within solvent-free melts. Here we describe the synthesis, properties and enzyme activity of self-contained reactive biofluids based on solvent-free melts of lipase-polymer surfactant nanoconjugates. Desiccated substrates in liquid (p-nitrophenyl butyrate) or solid (p-nitrophenyl palmitate) form can be mixed or solubilized, respectively, into the enzyme biofluids, and hydrolysed in the solvent-free state. Significantly, the efficiency of product formation increases as the temperature is raised to 150 °C. In aqueous environments, lipases catalyse the hydrolysis of fatty acid esters by a two-step mechanism that involves nucleophilic attack by a serine residue located within the active site to produce an acylated enzyme and alcohol product, followed by nucleophilic addition of a water molecule to liberate the fatty acid [1] . Conversely, in non-aqueous media, lipases can use other nucleophiles, such as methanol, to catalyse esterification and transesterification reactions [2] , [3] , [4] , [5] , [6] , [7] , [8] , [9] , [10] , [11] , [12] , [13] , although the explicit removal of water is not often a priority. Typically, enzyme reactions performed in organic solvents still contain a hydration layer at the surface of the protein, and the pervasiveness of the solvent in these examples highlights the requirement for a substrate delivery medium [14] , [15] , [16] , [17] , [18] , [19] , [20] , [21] , [22] , [23] , [24] , [25] . There have also been reports of lipase catalysis where the reaction proceeds with solvent quantities of one of the reagents [3] , [12] , [13] , where the lipases are typically present as either a lyophilized powder [12] , [13] , [26] , or immobilized on a substrate [2] , [3] , [8] , [10] , [27] , [28] , but there are no examples of molecularly dispersed enzymes catalysing reactions in the complete absence of a solvent. Previously, we reported on a novel method for the formation of solvent-free liquid proteins [29] , where the surfaces of the protein molecules were reengineered to display multiple copies of polymer surfactant molecules, which increased the range of the attractive intermolecular interactions to a distance that was commensurate with melting. Significantly, the room-temperature myoglobin biofluids contained significant levels of dynamic secondary and tertiary structure [30] , and remarkably, bound gaseous ligands such as carbon monoxide, sulphur dioxide, and oxygen reversibly in the complete absence of a solvent [31] . Although the persistent structure, function and dynamics exhibited by the solvent-free liquid myoglobin were remarkable, reversible gaseous oxygen binding could be considered a relatively primitive and robust biological process, which would occur provided that the haem prosthetic group was still present in the protein. Conversely, enzyme catalysis by a solvent-free liquid protein represents a considerable challenge, as the prerequisites for such a process include the correct conformation of the active site, and the presence of a medium for substrate and product mass transfer. Here we show for the first time that biologically active solvent-free liquid proteins can be prepared using lipases from the mesophile Rhizomucor miehei (RML) and thermophile Thermomyces lanuginosus (TLL). The lipases comprise an active site based around a serine-histidine-aspartate triad (Ser144-His257-Asp203 for RML, Ser146-His258-Asp201 for TLL) with substrate access regulated by conformational changes involving a helical ‘lid’ motif ( Fig. 1a ), and which together facilitate nucleophilic attack on the fatty acid ester substrate to produce the acylated enzyme and alcohol product ( Fig. 1b ). As a consequence, reaction in the solvent-free state requires substrate solubilization in the liquid enzyme, diffusion through the viscous melt, molecular access to the active site and conformational flexibility in the enzyme-polymer surfactant nanoconjugate. Moreover, turnover of the lipases requires nucleophilic addition of a water molecule to liberate the carboxylic acid ( Fig. 1b ), which should be effectively curtailed in the solvent-free phase. In light of these considerations, we demonstrate that the new lipase biofluids directly solubilize and hydrolyse short- or long-chain fatty acid esters from both the solid (p-nitrophenyl palmitate; pNPPal) and liquid ( p -nitrophenyl butyrate; pNPB) phase with limited substrate turnover. Significantly, the solvent-free liquid enzymes are extremely thermally stable, undergo re-folding from a half denaturation temperature of around 170 °C and, remarkably, exhibit increasing catalytic efficiency as the temperature is increased up to 150 °C. 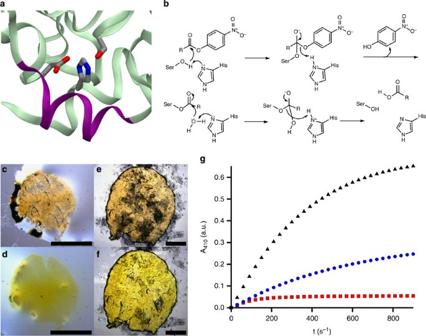Figure 1: Self-contained enzymatic biofluids. (a) Three-dimensional model showing the Ser144-His257-Asp203 catalytic triad of RML (PDB: 3TGL33) and helical ‘lid’ motif (purple loop). (b) Two-step mechanism for lipase-catalysed hydrolysis of pNPB (R=C3H7) or pNPPal (R=C15H31). (c–f) Optical microscopy images showing a mixture of the solvent-free liquid [C-RML][S1] and desiccated liquid pNPB substrate immediately after contact (c), and after incubation for 30 min at 80 °C (d), and a mixture of solvent-free liquid [C-RML][S1] and desiccated solid pNPPal immediately after contact (e) and after incubation for 24 h at 50 °C (f); scale bars, 800 μm. In both cases, development of the yellow colouration indicates lipase-catalysed formation of pNP in the solvent-free liquid enzymes. (g) Plot of time-dependent absorbance at 410 nm showing increase in pNP concentration with time demonstrating esterase activity in pNPB-containing solvent-free liquid [C-RML][S1] (black triangles), or [C-TLL][S1] (red squares) at 30 °C, and after incubating solvent-free liquid [C-RML][S1] at 110 °C for 1 h (blue circles). Figure 1: Self-contained enzymatic biofluids. ( a ) Three-dimensional model showing the Ser144-His257-Asp203 catalytic triad of RML (PDB: 3TGL [33] ) and helical ‘lid’ motif (purple loop). ( b ) Two-step mechanism for lipase-catalysed hydrolysis of pNPB ( R =C 3 H 7 ) or pNPPal ( R =C 15 H 31 ). ( c – f ) Optical microscopy images showing a mixture of the solvent-free liquid [C-RML][ S 1 ] and desiccated liquid pNPB substrate immediately after contact ( c ), and after incubation for 30 min at 80 °C ( d ), and a mixture of solvent-free liquid [C-RML][ S 1 ] and desiccated solid pNPPal immediately after contact ( e ) and after incubation for 24 h at 50 °C ( f ); scale bars, 800 μm. In both cases, development of the yellow colouration indicates lipase-catalysed formation of pNP in the solvent-free liquid enzymes. ( g ) Plot of time-dependent absorbance at 410 nm showing increase in pNP concentration with time demonstrating esterase activity in pNPB-containing solvent-free liquid [C-RML][ S 1 ] (black triangles), or [C-TLL][ S 1 ] (red squares) at 30 °C, and after incubating solvent-free liquid [C-RML][ S 1 ] at 110 °C for 1 h (blue circles). Full size image Solvent-free liquid lipase synthesis and characterization Viscous solvent-free liquid lipases were prepared using a three-step approach involving (i) preparation of cationized enzymes (C-RML and C-TLL), (ii) electrostatic coupling of the anionic polymer surfactants poly(ethylene glycol) 4-nonylphenyl 3-sulfopropyl ether ( S 1, ) or carboxylated Brij-L23 ( S 7 ) ( Supplementary Fig. 1 ) to C-RML and C-TLL, to produce aqueous protein-polymer surfactant constructs ([C-RML][ S 1 ], [C-RML][ S 7 ], [C-TLL][ S 1 ] and [C-TLL][ S 7 ]) that were ca. 2–3 nm larger in hydrodynamic diameter than the respective native proteins ( Supplementary Fig. 2 ), and (iii) extensive lyophilization of the aqueous constructs followed by thermal annealing at 65 °C ( Supplementary Information , Materials and Methods). Differential scanning calorimetry traces from the solvent-free liquid lipases showed reversible endothermic melting transitions at 25 °C and 44 °C, or 26 °C and 46 °C for [C-RML][ S 1 ] and [C-RML][ S 7 ], or [C-TLL][ S 1 ], and [C-TLL][ S 7 ], respectively ( Supplementary Fig. 3 ), which were different from values determined for the neat polymer surfactants ( S 1 =31 °C; and S 7 =36 °C). Thermogravimetric analysis of the solvent-free protein liquids gave water contents ranging from 0.3 to 0.6 wt% ( Supplementary Fig. 4 ), which was equivalent to 20–30 water molecules per construct. This was more than an order of magnitude lower than the number of water molecules required to cover the solvent-accessible surface area of the enzymes (1,300 and 1,250 for RML and TLL, respectively), and significantly lower than the accepted water content required for enzymatic activity (20–40 wt%) [32] . Esterase activity in a solvent-free environment A series of assays were developed to test for esterase activity in the solvent-free liquid lipases. We introduced small quantities of anhydrous liquid pNPB or desiccated solid pNPPal substrates directly into the solvent-free liquid lipases prepared at just above the melting temperatures ( Supplementary Information , Materials and Methods). Significantly, addition of the liquid or the pNPPal waxy solid to each of the four solvent-free liquid lipases resulted in the development of an intense yellow colour that was distributed throughout the enzyme-polymer surfactant melt, signifying the formation of the p -nitrophenol (pNP) product ( Fig. 1c–f ). These observations were intriguing for several reasons. First, they showed that desiccated substrates in either liquid or solid form could be effectively introduced into the solvent-free liquid lipases, indicating that the biofluid phase boundary was accessible to auxiliary agents either by liquid–liquid miscibility or solubilization at the liquid–solid interface. We attribute this behaviour to the amphiphilic nature of the polymer surfactant corona, which presents a dielectric medium that is compatible with the relatively hydrophobic substrate molecules. Significantly, control experiments performed using neat desiccated surfactant showed slow dissolution of pNPPal over time ( Supplementary Fig. 5 ). Second, mass transfer of the substrates was possible in the viscous enzyme melt, and although diffusion was slow at temperatures just above the melting temperatures, this was sufficient to distribute the molecules throughout the solvent-free liquid phase. Third, the lipases remained accessible to substrate recognition even though the enzyme molecules were incarcerated in a corona of polymer surfactant chains, suggesting that the helical lid motif could still sample catalytically competent conformations or was permanently open, and that the polymer surfactant shell was permeable to small molecules. In this regard, synchrotron radiation small angle X-ray scattering profiles from the solvent-free [C-RML][ S 1 ] and [C-TLL][ S 1 ] liquids at 30 °C showed protein–protein correlation peaks at 0.104 Å −1 and 0.106 Å −1 ( Supplementary Fig. 6 ). These values corresponded to respective centre-to-centre separation distances of 60 and 59 Å, and in both cases were consistent with a structural model based on a globular protein core (RML and TLL have molecular dimensions of approximately 45 × 45 × 40 Å (refs 33 , 34 ), surrounded by a condensed polymer surfactant corona with a shell thickness of approximately 10 Å. Significantly, the yellow colouration observed in the optical microscopy images confirmed that binding of the substrates to the lipases was associated with bond cleavage, indicating that the enzymes remained functional in the solvent-free melt, and suggesting that the protein secondary structure and local configuration of the Ser-His-Asp triad at the active site were not significantly perturbed in the solvent-free biofluids. We tested the latter assumption by recording synchrotron radiation circular dichroism (SRCD) spectra on solvent-free samples of liquid [C-RML][ S 7 ] and [C-TLL][ S 7 ] ( Supplementary Fig. 7 ). In both cases, deconvolution of the SRCD spectra showed high levels of secondary structure ( Table 1 ), in agreement with attenuated total reflection Fourier transform infrared spectroscopy data ( Supplementary Fig. 8 ). The secondary structure distribution of the solvent-free liquid [C-RML][ S 7 ] was almost identical to that of the aqueous RML precursor, although a reduction in the α-helical content was observed for solvent-free liquid [C-TLL][ S 7 ] compared with native TLL. Table 1 Estimated secondary structure contents. Full size table Ultraviolet–visible spectroscopy in transmission mode was used to assay the lipase activity of the solvent-free [C-RML][ S 1 ] and [C-TLL][ S 1 ] liquids by monitoring the rate of formation of pNP ( ε 410 =18.3 mM −1 cm −1 ) from pNPB at 30 °C ( Fig. 1g ). 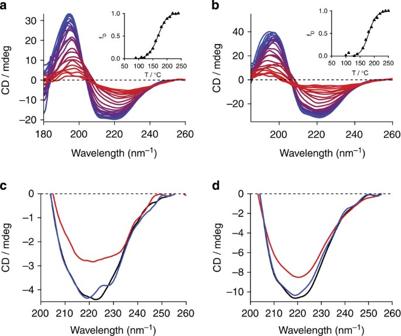Figure 2: Secondary structure stabilization and refolding in solvent-free liquid lipases. Far-ultraviolet SRCD spectra from solvent-free liquids of [C-RML][S7] (a) and [C-TLL][S7] (b) over a temperature range of 0–250 °C (blue to red profiles) at 10 °C intervals. Insets show fraction of denatured secondary structure as a function of temperature and resulting sigmoidal fits (solid lines). The CD intensity at 222 nm was used as an order parameter. Far-ultraviolet SRCD spectra showing highly efficient unfolding and refolding (≥95%) after heating samples of solvent-free liquid [C-RML][S7] (c) or [C-TLL][S7] (d) from 50 (black curve) to 150 °C (red curve), followed by cooling to 50 °C at a rate of 100 °C min−1(blue curve). The initial rates of pNP formation by the [C-RML][ S 1 ] and [C-TLL][ S 1 ] biofluids were estimated at 0.04±0.01 and 0.02±0.007 μmol min −1 mg −1 ( Table 2 ), respectively, which suggested that the mesophile-derived [C-RML][ S 1 ] biofluid was more effective at physiological temperatures. Control inhibition experiments using the serine protease inhibitor phenylmethanesulfonyl fluoride (PMSF) gave a significant reduction in the lipase activity (≈6-fold) of the [C-RML][ S 1 ] biofluid with pNPB ( Supplementary Fig. 9 ), which signified that the activity was associated with the Ser-His-Asp triad at the active site. It is possible that that partitioning of PMSF into the hydrophobic domains of the polymer surfactant corona reduced the efficacy of the inhibitor, although limited hydrolysis of the pNPB from an increase in the nucleophilicity of surface residues in the solvent-free state could not be ruled out. The initial rates of the uninhibited lipase biofluids were significantly lower than those determined for the respective aqueous native, cationized or conjugated proteins at 37 °C ( Table 2 and Supplementary Figs 10 and 11 ). This reduction in rate was attributed to the large resistance to substrate and product mass transfer arising from the high viscosity of the biofluids. Table 2 Enzyme activities of the solvent free liquid lipases. Full size table Given the very low water content of the solvent-free liquid lipases, it seems plausible that the low threshold absorbance values observed in the ultraviolet–visible spectroscopy profiles were associated with limited turnover of the two-step cycle such that a large population of acylated enzymes were present in the solvent-free medium ( Fig. 1g ). Significantly, analysis of the spectroscopic assay for the [C-RML][ S 1 ]/pNPB biofluid gave a turnover number of 6±2, indicating that in the solvent-free liquid state RML was able to use some of the limited number of local water molecules (20–30 per construct) present in the mixture. To test this hypothesis, solvent-free liquid [C-RML][ S 1 ] was incubated at 110 °C for 1 h to further reduce the sub-solvation water content, and the assay repeated ( Fig. 1g ). This resulted in a reduction of the turnover number to 1.4±0.4, which, in the absence of thermal deactivation (see below), indicated that the [C-RML][ S 1 ] conjugate could use the limited number of water molecules to complete the reaction cycle via nucleophilic addition to the acylated enzyme intermediate. In contrast, there was no evidence of turnover from the [C-TLL][ S 1 ]/pNPB assay, which signified that the reaction stopped after enzyme acylation. The active site of the thermophile-derived TLL is highly constrained [35] when compared with other lipases such as RML, which has a shallow-bowl conformation with a large open cavity [36] . Accordingly, the difference in the active site geometries could be responsible for the inability of the TLL biofluid to use the limited water molecules available in the solvent-free liquid. Enzyme activity at extreme temperatures Given the hyperthermophilic behaviour previously observed for solvent-free liquid proteins prepared from cationized myoglobin [37] or lysozyme [38] , we established a series of experiments to ascertain the thermal stability and refolding properties of the lipase melts to determine whether enzyme activity in the solvent-free liquid state could be maintained over an extended temperature range. We first used temperature-dependent SRCD spectroscopy to probe the equilibrium thermal denaturation pathways of solvent-free liquid [C-RML][ S 7 ] and [C-TLL][ S 7 ] over a temperature range of 0 to 250 °C ( Fig. 2a,b ). 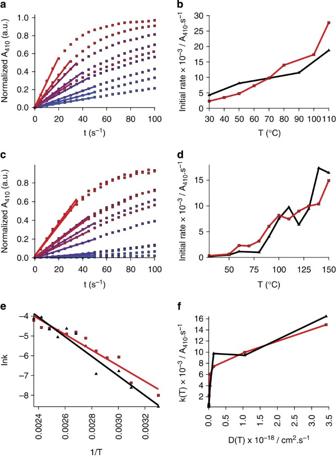Figure 3: Temperature-dependent esterase activity in solvent-free liquid lipases. (a) Plots of absorbance (diffuse reflectance) at 410 nm against time showing increase in the initial rate of formation of pNP from pNPB by solvent-free liquid [C-TLL][S1] over a temperature range of 30 (blue) to 110 °C (red) at 10 °C intervals. (b) Plot of initial rate of reaction of pNPB with solvent-free liquid [C-RML][S1] (black triangles) and [C-TLL][S1] (red squares) as a function of temperature. (c) Plots of diffuse reflectance ultraviolet–visible spectroscopy absorbance at 410 nm against time showing an increase in initial rate with temperature for the reaction between pNPPal and solvent-free liquid [C-RML][S1] over a temperature range of 50 (blue) to 150 °C (red) at 10 °C intervals. (d) Plot showing an increase in the initial rate with temperature for the reaction between pNPPal and solvent-free liquid [C-RML][S1] (black triangles) or solvent-free liquid [C-TLL][S1] (red squares). (e) Arrhenius plots ofln k(wherekis the temperature-dependent initial rate) against 1/Tfor the reaction between pNPPal and solvent-free liquid [C-RML][S1] (black triangles) or [C-TLL][S1] (red squares). (f) Plot of temperature-dependent initial rate of reaction [k(T)] between pNPPal and solvent-free liquid [C-RML][S1] as a function of the temperature-dependent Stokes–Einstein diffusion coefficient [D(T)] (see equation 6 inSupplementary Methods). Significantly, both biofluids exhibited extreme hyperthermophilic behaviour with half denaturation temperatures ( T m ) of 168 °C and 180 °C, respectively ( Table 3 and Fig. 2c ), which were ~100 °C higher than their aqueous [C-RML][ S 7 ] and [C-TLL][ S 7 ] precursors ( Table 2 and Supplementary Figs 12 and 13 ), and reflected their respective meso- and thermophilic origins. Moreover, highly efficient refolding (≥95%) was evident when cooling from temperature as high as 150 °C ( Fig. 2d,e ). Thermal denaturation thermodynamics (see Supplementary Materials and Methods , Equilibrium Thermodynamics) were used to evaluate the free energy of denaturation ( ΔG D , Supplementary Fig. 14 ) and the change in entropy ( ΔS m ) and enthalpy ( ΔH m ) at the half denaturation temperature ( T m ) ( Table 3 ). The data indicated that thermal stabilization was predominately associated with a reduction in ΔS m and not via a significant increase in ΔH m. , which was consistent with either a relatively less disordered compact denatured state, or a more disordered native state [37] . The former seems more probable given the high levels of secondary structure and the highly crowded environment of the solvent-free liquid phase across a temperature range of 30 to 150 °C. Figure 2: Secondary structure stabilization and refolding in solvent-free liquid lipases. Far-ultraviolet SRCD spectra from solvent-free liquids of [C-RML][ S 7 ] ( a ) and [C-TLL][ S 7 ] ( b ) over a temperature range of 0–250 °C (blue to red profiles) at 10 °C intervals. Insets show fraction of denatured secondary structure as a function of temperature and resulting sigmoidal fits (solid lines). The CD intensity at 222 nm was used as an order parameter. Far-ultraviolet SRCD spectra showing highly efficient unfolding and refolding (≥95%) after heating samples of solvent-free liquid [C-RML][ S 7 ] ( c ) or [C-TLL][ S 7 ] ( d ) from 50 (black curve) to 150 °C (red curve), followed by cooling to 50 °C at a rate of 100 °C min −1 (blue curve). Full size image Table 3 Thermodynamic parameters for solvent-free liquid lipases. Full size table In light of these results, we used diffuse reflectance (DR) ultraviolet–visible spectroscopy to monitor the temperature dependence of the rate of pNP formation in pNPB-containing solvent-free liquid lipases ( Fig. 3a and Supplementary Fig. 15 ). Significantly, an increase in the temperature resulted in a rate enhancement for all of the solvent-free liquid lipases. For example, increasing the temperature from 30 to 110 °C gave a 4-fold and 12-fold rate increase in the [C-RML][ S 1 ] and [C-TLL][ S 1 ] solvent-free reaction fluids, respectively ( Fig. 3b ), which was consistent with the thermophilic origin of the TLL-base enzyme-polymer surfactant construct. Moreover, incubation of the [C-RML][ S 1 ] melt for 1 h at 150 °C followed by cooling to 30 °C showed almost complete retention of the enzymatic activity when pNPB was added ( Supplementary Fig. 16 ), consistent with the almost complete refolding of the lipase under these conditions. In contrast, control experiments undertaken in pNPB-containing aqueous solutions at 85 °C showed negligible enzyme activity in the lipase-polymer surfactant constructs ( Supplementary Fig. 17 ). Figure 3: Temperature-dependent esterase activity in solvent-free liquid lipases. ( a ) Plots of absorbance (diffuse reflectance) at 410 nm against time showing increase in the initial rate of formation of pNP from pNPB by solvent-free liquid [C-TLL][ S 1 ] over a temperature range of 30 (blue) to 110 °C (red) at 10 °C intervals. ( b ) Plot of initial rate of reaction of pNPB with solvent-free liquid [C-RML][ S 1 ] (black triangles) and [C-TLL][ S 1 ] (red squares) as a function of temperature. ( c ) Plots of diffuse reflectance ultraviolet–visible spectroscopy absorbance at 410 nm against time showing an increase in initial rate with temperature for the reaction between pNPPal and solvent-free liquid [C-RML][ S 1 ] over a temperature range of 50 (blue) to 150 °C (red) at 10 °C intervals. ( d ) Plot showing an increase in the initial rate with temperature for the reaction between pNPPal and solvent-free liquid [C-RML][ S 1 ] (black triangles) or solvent-free liquid [C-TLL][ S 1 ] (red squares). ( e ) Arrhenius plots of ln k (where k is the temperature-dependent initial rate) against 1/ T for the reaction between pNPPal and solvent-free liquid [C-RML][ S 1 ] (black triangles) or [C-TLL][ S 1 ] (red squares). ( f ) Plot of temperature-dependent initial rate of reaction [ k(T) ] between pNPPal and solvent-free liquid [C-RML][ S 1 ] as a function of the temperature-dependent Stokes–Einstein diffusion coefficient [ D(T )] (see equation 6 in Supplementary Methods ). Full size image To test the efficacy of the lipase biofluids at higher temperatures, pNPB (boiling point, ca. 125 °C) was replaced with the less volatile pNPPal, and the range of temperature-dependent assays extended to 150 °C ( Fig. 3c and Supplementary Fig. 18 ). Control DR ultraviolet–visible spectroscopy experiments performed on pNPPal from 30 to 150 °C showed negligible decomposition ( Supplementary Fig. 19 ) and differential scanning calorimetry gave a melting temperature of 66 °C ( Supplementary Fig. 20 ). Remarkably, increasing the temperature up to a maximum of 150 °C resulted in a constant increase in the rate of pNPPal hydrolysis for all four lipase biofluids. Specifically, increasing the temperature from 30 to 150 °C resulted in an 88-fold and 45-fold increase in initial rate for [C-RML][ S 1 ] and [C-TLL][ S 1 ], respectively ( Fig. 3d ). Interestingly, there was no sudden increase in the initial rates when the temperature was increased beyond the melting temperature of pNPPal, which confirmed that the solvent-free liquids solubilized the solid substrate effectively. The persistent activity of the solvent-free lipases at extreme temperatures was remarkable and correlated well with the hyperthermal stability of the biofluid structures. The temperature-dependent increase in the rate of hydrolysis of pNPB and pNPPal is likely to be extremely complex, involving contributions from the increase in k T (Arrhenius behaviour), as well as from temperature-induced reduction in viscosity, leading to increased substrate and product diffusion rates. Plots of ln k (where k is the experimentally determined initial rate) versus 1/ T were calculated from the solvent-free liquid [C-RML][ S 1 ]/pNPPal assay rate data and showed a linear response ( Fig. 3e ), highly consistent with Arrhenius behaviour. Temperature-dependent rheometry experiments performed on the [C-RML][ S 1 ] biofluid indicated that the estimated Stokes–Einstein diffusion coefficient ( D ) for pNPPal increased by ca. 1,800-fold from 1.9 × 10 −21 to 3.4 × 10 −18 cm 2 s −1 as the temperature was increased from 30 to 150 °C ( Supplementary Fig. 21 and see Supplementary Methods ), which would also favour an increase in initial reaction rate. Plots of temperature-dependent reaction rate against the temperature-dependent diffusion coefficient of pNPPal yielded a non-linear relationship over the entire temperature range ( Fig. 3f ), indicating that although the decrease in viscosity could not be completely ruled out, increases in k B T rather than a predominantly diffusion-only mechanism (rate proportional to the D with respect to temperature) was the predominant cause of the increased enzyme activity in the heat-treated solvent-free biofluids. In conclusion, we have shown the unprecedented formation and characterization of solvent-free liquid lipases from RML and TLL, which are functional self-contained biofluids that can directly solubilize substrates and catalyse reactions. We have demonstrated that the hyperthermophilic behaviour of the protein structures directly translates to the ability to not only perform reactions at temperatures as high as 150 °C, but with increasing efficiency. The results demonstrate that even in the absence of a solvent, the polymer surfactant corona surrounding the enzymes stabilizes the enzyme structure and acts as a continuum for the delivery of substrate molecules to the active site. The ability to produce reactive enzymatic biofluids that can function at extreme temperatures and directly solvate and convert substrates should provide new directions in industrial catalysis and bionanotechnology. Activity assays Enzyme activity assays were performed on the solvent-free liquid lipases by monitoring the rate of formation of pNP at 410 nm ( ε 410 =18.3 mM −1 cm −1 ) from pNPB (Sigma, UK) or pNPPal using ultraviolet–visible spectroscopy. To promote the formation of the p -nitrophenolate chromophore, the aqueous lipase-polymer surfactant conjugates were adjusted to pH 8 using small quantities of TRIS buffer before lyophilization and melting. Solvent-free liquid assays performed just above the melting temperatures of the enzyme-polymer surfactant solids (30 °C and 45 °C for the S 1 and for the S 7 formulations, respectively) were undertaken by spreading 3.4±0.2 mg of liquid [C-RML][ S 1 ], [C-TLL][ S 1 ], [C-RML][ S 7 ] or [C-TLL][ S 7 ] over a 2 cm 2 area on one face of a two-part quartz cell (0.01 mm path length), followed by addition of 2 μl of desiccated pNPB. The quartz cell was immediately sealed with polytetrafluoroethylene tape and the increase in absorbance at 410 nm measured at 5 s intervals for 15 min using a Perkin Elmer Lambda 25 ultraviolet–visible spectrometer fitted with a PTP-6 peltier control unit. For high-temperature assays (≤150 °C), samples were prepared as above and then raised to increasing temperatures, typically at 10 °C intervals at a rate of 10 °C min −1 , with 30 s equilibration before measurements. The absorbance at 410 nm was monitored at the given temperatures at 5 s intervals for 15 min using a Perkin Elmer Lambda 35 ultraviolet–visible spectrometer equipped with a Labsphere DR accessory fitted with a custom-made reflective thermal stage. For enzyme activity assays involving solid pNPPal, 3 mg aliquots of desiccated pNPPal powder were introduced directly to the solvent-free lipase liquids and sealed within the synthetic quartz cell with polytetrafluoroethylene tape as described above. Diffuse reflectance spectroscopy was used as reliable transmission measurement could not be made due to scattering from the solid substrate. Activity assay data analyses Enzyme activities of the solvent-free lipase liquids against pNPB at 30 °C were evaluated from averaged ( n =>5) initial reaction rates using linear regression analysis of the ultraviolet–visible spectroscopy data (transmission, 0.01 mm path length). Turnover values were estimated based on the absorbance values at 410 nm obtained for the completed reaction (averages of n =>5). This was achieved by dividing the pNP concentration ( ε 410 =18.3 mM −1 cm −1 ) by the active site concentration (that is, concentration of lipase in the solvent-free liquid). Concentrations of the enzyme and substrate within the mixtures were calculated from constituent mass fractions, using densities of 1.35 and 1.2 g cm −3 for lipase and pNPB, respectively. Temperature-dependent enzyme activities were evaluated from the initial rates obtained by plotting A 410 against time at various temperatures, and the data were normalized after fitting using an exponential function to mitigate variations in absolute absorbances arising from variable path lengths in the diffuse reflectance measurements. The resultant plots of rate against temperature were expressed as the natural log of the initial rate (ln k ) against reciprocal temperature (1/ T ), where linear plots indicate Arrhenius behaviour. Thermal cycle assays were performed on solvent-free liquid [C-RML][ S 1 ] to study the effect of water removal and involved incubating the sample at 110 °C for 1 h. This equilibration period was established via analogous thermogravametric analysis experiments ( Supplementary Information and Supplementary Fig. 4b ), which showed no further mass loss at 110 °C after 1 h. Esterase inhibition assays Lipase inhibition control experiments were performed on the solvent-free [C-RML][ S 1 ] liquid at 30 °C via the addition of the serine protease inhibitor PMSF to the aqueous [C-RML][ S 1 ] precursor, followed by lyophilization and melting to give a final mass fraction of 10 wt%. Control activity assays were preformed on aqueous RML, C-RML, [C-RML][ S 1 ], TLL, C-TLL and [C-TLL][ S 1 ] at nmol concentrations with 0.36 mM pNPB in 50 mM TRIS buffer (pH 8) at 37 °C. Absorbance at 410 nm was monitored at 5 s intervals for 3 min using a Perkin Elmer Lambda 25 ultraviolet–visible spectrometer fitted with a PTP-6 peltier control unit. In all cases, enzyme activity was normalized to the rate of pNPB degradation observed in the absence of the enzymes and presented as the average of >5 repeats. General details on the synthesis procedures and characterization techniques have been deposited as Supplementary Information . How to cite this article: Brogan, A. P. S. et al . Enzyme activity in liquid lipase melts as a step towards solvent-free biology at 150 °C. Nat. Commun. 5:5058 doi: 10.1038/ncomms6058 (2014).